Self-assembly of colloid-cholesteric composites provides a possible route to switchable optical materials Colloidal particles dispersed in liquid crystals can form new materials with tunable elastic and electro-optic properties. In a periodic ‘blue phase’ host, particles should template into colloidal crystals with potential uses in photonics, metamaterials and transformational optics. Here we show by computer simulation that colloid/cholesteric mixtures can give rise to regular crystals, glasses, percolating gels, isolated clusters, twisted rings and undulating colloidal ropes. This structure can be tuned via particle concentration, and by varying the surface interactions of the cholesteric host with both the particles and confining walls. Many of these new materials are metastable: two or more structures can arise under identical thermodynamic conditions. The observed structure depends not only on the formulation protocol but also on the history of an applied electric field. This new class of soft materials should thus be relevant to design of switchable, multistable devices for optical technologies such as smart glass and e-paper. When spherical colloidal particles are mixed into a nematic liquid crystal, they disrupt the orientational order in the fluid and create defects (disclination lines) in the nematic close to their surfaces. To minimize the free-energy cost, it is generally advantageous for defects to be shared: therefore, the colloidal particles have a generic tendency to aggregate. Such aggregates may further self-assemble into lines [1] , 2D crystals [2] , planar structures [3] or 3D amorphous glasses [4] . Besides being of fundamental interest to material science, these structures may have tunable elastic and optical properties [5] . Hence they offer exciting prospects for applications as biosensors [6] or as new devices [7] , [8] . However, one may also choose to disperse colloidal particles in a cholesteric, rather than nematic, liquid crystal. The molecules making up this material are chiral, and this causes their average orientation (described by a director field) to rotate in space in a helical manner, rather than remain uniform as in nematics. This typically creates a 1-dimensional periodic structure, called the cholesteric phase, whose wavelength is the pitch, p . The periodicity can, however, become fully three-dimensional (3D) in the so-called blue phases (BPs) [9] . BPs arise because the director field can twist around more than one direction at once (see the cartoon in Supplementary Fig. 1 ). Such double twist regions (generally cylinders) are energetically favoured at high enough molecular chirality, but lead to geometric frustration because it is impossible to tile the whole 3D space with double twist cylinders without also introducing ‘disclination lines’. (These are singular topological defects on which the director field is undefined.) In BPs, these disclination lines themselves either form a 3D periodic regular lattice (in so called BPI and BPII) or remain disordered (BPIII) [10] . BPs are stabilised by the tendency of chiral molecules to twist, but destabilised by the cost of forming topological defects (which locally diminish the molecular alignment). In conventional cholesteric materials [9] , this balance is only achievable in a narrow temperature range of a few degrees, around the onset of liquid crystalline ordering. However, recent advances in formulation have widened this stability range enormously [11] , [12] , [13] , [14] . Most recently, templated BPs with a stability range of −125 to 125 °C have been reported [15] , paving the way to applications of BPs in operational display devices. Besides being remarkable materials in themselves, BPs offer significant promise as hosts for dispersing colloidal particles. Because BPs contain a disclination network even in the absence of particles, they can potentially template colloidal self-assembly. This was proved recently by simulations of BP-dispersed nanoparticles that exclude the surrounding liquid crystal but otherwise have negligible surface interaction with it (to give a so-called ‘weak anchoring’ regime) [16] , [17] . Such particles are attracted to the disclination network in BPs: by covering up the defect cores, the high elastic energy cost of those regions is avoided. The pre-existing order of the defect network then templates particles into a regular colloidal crystal of the same periodicity. Because this structure has a wavelength in the visible range, the resulting material should inherit (and probably enhance) the incomplete photonic bandgap of the parent BP, as exploited for instance in laser devices [12] ; for related possibilities see ref. 18 . A second compelling reason to study colloidal-BP composites is that, even without particles, BPs can show several competing metastable free-energy minima, corresponding to different topologies of the defect network [19] , [20] , with a strong dependence on applied electric or magnetic fields [21] . Adding particles is likely to further enrich the free-energy landscape, creating composites that might be promising candidates for bistable or multistable devices, in which energy is needed only to switch optical properties and not to maintain them. (This is the e-paper paradigm [22] and can lead to huge energy savings.) To explore such metastability, and switching strategies between states, we require multi-unit-cell, time-dependent simulations. These go beyond previous studies of colloidal-BP composites [17] but follow comparable simulations of pure BPs [10] , [21] , [23] , and isolated and dimeric colloidal particles in cholesterics [24] , [25] . The simulations presented here are representative of a liquid crystal BP with unit cell size in the range of 100–500 nm (ref. 9 ) and particles with a diameter of around 50 nm. The simulations address both the bulk structure, and the structure that forms when the colloidal dispersion is confined in a narrow sandwich of width comparable to the unit cell size [26] . It is seen that a wide variety of structure is possible and may be influenced by parameters including the solid volume fraction and the details of the anchoring at the colloid surface (and the at the surface of the confining walls). Further, evidence is found for metastable switching of this structure in an applied electric field. Details of the computational approach are set out in the Methods section, while simulation parameters are reported in the Supplementary Methods . Structure in bulk BPI We show in Fig. 1a–d the final state structures of four simulations in which we first equilibrated a stable BPI disclination network in bulk (with periodic boundary conditions) and then dispersed colloidal particles at random within it. Among dimensionless control parameters are the particle solid volume fraction ϕ ( ϕ =1% or 5%); the ratio of particle radius to the BP lattice parameter (here ) and the ratio w = WR / K where W is the anchoring strength of the cholesteric at the particle surface and K is the elastic constant of the liquid crystal. The anchoring strength is defined such that W >0 imparts a preferred orientation to the director field at the particle surface. This orientation can be either normal to the surface or in a plane tangential to the surface, a property related to surface chemistry in experimental systems. We choose w =0.23, 2.3 that are within typical experimental range [4] . This parameter can be viewed as the ratio of the anchoring energy, WR 2 , to the elastic energy scale for distortion KR . 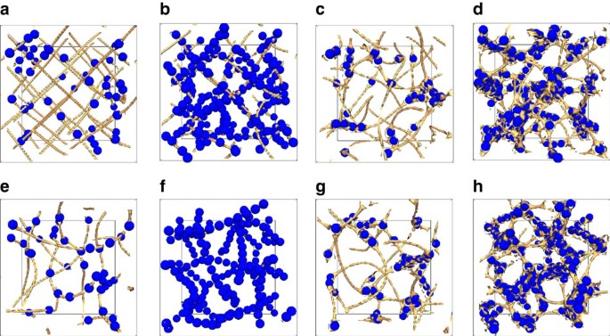Figure 1: Bulk blue phase structures. Snapshots of the states obtained after dispersing a suspension of colloidal nanoparticles within a cholesteric liquid crystal in the BPI-forming region.a–dcorrespond to the case of a dispersion of particles in a pre-equilibrated BPI phase;e–hare obtained by dispersing colloids in an isotropic phase and then quenching into the range where BPI is stable, leading to the formation of an amorphous, BPIII-like, disclination network. Structures correspond to (a) and (e)w=0.23 andϕ=1%; (b) and (f)w=0.23 andϕ=5%; (c) and (g)w=2.3 andϕ=1%; (d) and (h)w=2.3 andϕ=5%. The anchoring of the director field to the colloidal surface is normal. (For the full parameter list used to generateFigs 1,2,3seeSupplementary Notes.) For clarity, only a portion of the simulation box is shown its linear extent being(one-eighth of the total volume); the full structures are shown inSupplementary Figs 2 and 3. Figure 1: Bulk blue phase structures. Snapshots of the states obtained after dispersing a suspension of colloidal nanoparticles within a cholesteric liquid crystal in the BPI-forming region. a – d correspond to the case of a dispersion of particles in a pre-equilibrated BPI phase; e – h are obtained by dispersing colloids in an isotropic phase and then quenching into the range where BPI is stable, leading to the formation of an amorphous, BPIII-like, disclination network. Structures correspond to ( a ) and ( e ) w =0.23 and ϕ =1%; ( b ) and ( f ) w =0.23 and ϕ =5%; ( c ) and ( g ) w =2.3 and ϕ =1%; ( d ) and ( h ) w =2.3 and ϕ =5%. The anchoring of the director field to the colloidal surface is normal. (For the full parameter list used to generate Figs 1 , 2 , 3 see Supplementary Notes .) For clarity, only a portion of the simulation box is shown its linear extent being (one-eighth of the total volume); the full structures are shown in Supplementary Figs 2 and 3 . Full size image For a single colloidal particle in a nematic fluid, w controls the formation of a local topological defect at the particle surface [5] , with weak distortion of the nearby fluid at small w . In the colloidal-BP system, w also plays a determining role in the final composite structure. When w is small ( Fig. 1a,b ; Supplementary Movies 1 and 2 ), the attraction of particles to the disclination lattice causes the lattice to become covered by particles, with little disruption of its long-range order. Thus, a templated colloidal crystal is created, as first reported in ref. 17 . Interestingly, the weak but finite anchoring apparently creates an elastic force between the colloidal particles, which leads to very slow dynamics ( Supplementary Fig. 4 ) and the formation of small colloidal lines within disclinations, especially for dilute samples ( Fig. 1a ). It seems likely that polymer-stabilized BPs [11] work by a similar principle to this small w case, with a weak segregation of monomers towards the defect regions. For large w ( Fig. 1c,d ; Supplementary Movies 3 and 4 ), the picture changes markedly. Each colloidal particle now disrupts significantly the order of the nearby fluid, with defect formation close to its surface [5] . The resulting strong disruption of local liquid crystalline order around each particle leads now to a strong interparticle attraction. This restructures the disclination network completely, destroying the long range order of the original BPI topology. Most notably, particle aggregation favours the formation of defect junctions, where four disclinations meet. This structural motif is present in the unit cell of BPII rather than BPI (and also seen in the amorphous BPIII (ref. 10 )). The particle clusters are disjoint at low volume fractions ( ), but they interact elastically via the connecting disclinations. At larger ϕ , the aggregates join up to form a percolating colloidal cluster, which essentially templates the disclinations rather than vice versa. As colloidal-nematic composites [4] , all the structures in Fig. 1a–d should be soft solids, of nonzero elastic modulus G at low frequency. This contrasts with pure BPs, where G =0 as the fluid can flow with a finite viscosity via permeation of molecules through a fixed defect lattice [27] , [28] . We expect the structures in Fig. 1a–c to be only weak gels, as here the defect network percolates but particle contacts do not. This is broadly similar to the cholesteric-nanoparticle gel reported in ref. 29 (with G <1 Pa). In contrast, the colloidal gel structure in Fig. 1d should be much more resistant mechanically, due to the formation of a thick percolating particle network. The structure is now akin to that of the self-quenched glass found in colloidal-nematic composites [4] at much higher volume fraction (over 20% as opposed to below 5% here), for which G~10 3 Pa. This figure is consistent with an estimate obtained by comparing the mechanical properties of the network of defects stabilized by colloidal particles with those of rubber [30] for the relevant simulation parameters (see Supplementary Table 1 ). A more practical protocol for including particles in a BPI phase is to disperse the particles at random in an isotropic phase and then quenching this into the temperature range where BPI is stable. Here we know that, without particles, the kinetics can favour disordered (BPIII-like) intermediates, which may be long lived or even metastable [23] . Figure 1e–h shows outcomes of such a quench protocol with the same parameter sets as in Fig. 1a–d . For small w , the particles again decorate the disclination lines, but are this time templated onto an amorphous network rather than an ordered one. Increasing the volume fraction ( Fig. 1f ) leads to a more even coverage with a better defined particle spacing. In contrast, for large w , strong interparticle forces again dictate the self-assembly. At low concentrations, discrete particle clusters decorate an amorphous defect lattice ( Fig. 1g ), whereas at higher ϕ a percolating network of colloidal strands (the gel in Fig. 1h ) is again seen. The structures in Fig. 1a–h have been followed for ~20 ms (see Supplementary Fig. 4 ); they correspond to either very slowly evolving states or deep metastable minima (elastic interactions are of order KR and dwarf thermal motion, see Supplementary Fig. 4 and refs 5 , 18 ). It may be possible to anneal the structures obtained via the quench route, although we have not attempted this in simulation. The results presented suggest that even when starting with colloidal particles randomly dispersed in an ordered BP, the particles are able to distort the structure ( Fig. 1a,b ). This suggests that it would be difficult to identify a quench protocol which would lead to less, rather than more, disorder. Structures in confined BPI In display devices and other optical applications, it is typical for liquid crystals to be strongly confined (and subject to strong boundary effects), in contrast to the bulk geometries considered above. We therefore next describe how colloidal suspensions self-assemble in thin sandwiches (thickness ), whose confining walls can favour either tangential (planar degenerate) or normal (homeotropic) orientation of the director field. For simplicity, we here impose one or the other as a strict boundary condition. 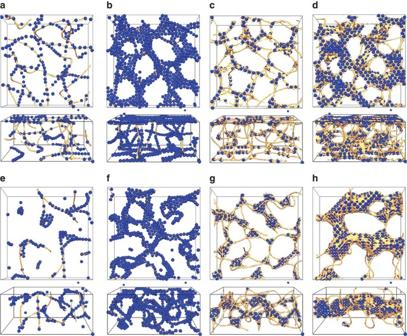Figure 2: Confined blue phase structures. Snapshots of the steady states obtained when a dispersion of colloids in the isotropic phase is placed in a sandwich geometry and then quenched into a regime where BPI is stable in the bulk. Both top and side views are provided. The anchoring of the director field at the walls is normal fora–dand planar fore–h. Structures correspond to (a) and (e)w=0.23 andϕ=1%; (b) and (f)w=0.23 andϕ=4%; (c) and (g)w=2.3 andϕ=1%; (d) and (h)w=2.3 andϕ=4%. As inFig. 1, only one quarter of the simulation box is shown for clarity (its horizontal extent beingand vertical extentin the narrow direction); the full structures are shown inSupplementary Figs 5 and 6. Figure 2a–d shows the case of normal wall anchoring on varying ϕ and w . We quench from the isotropic to the ordered phase as was done in Fig. 1e–h , and again find a metastable, amorphous disclination network (see Supplementary Methods ). The resulting colloidal-cholesteric composites are somewhat similar to those seen in the bulk: for small w the particles are templated by the network ( Fig. 2a,b ), whereas for large w we observe isolated clusters ( Fig. 2c ) and percolated colloidal gels ( Fig. 2d ), for ϕ =1 and 4%, respectively. There are, however, significant effects of the confining walls. First, the normal anchoring at the wall recruits particles there, giving (for the chosen h ) a density enhancement of the colloid particles at both walls (see side-views in Fig. 2a–d ). Second, the clusters formed at large w are themselves anisotropic with an oblate habit. These clusters are similar to those reported experimentally for large colloid particles in a cholesteric (but non-BP) host [31] . Figure 2: Confined blue phase structures. Snapshots of the steady states obtained when a dispersion of colloids in the isotropic phase is placed in a sandwich geometry and then quenched into a regime where BPI is stable in the bulk. Both top and side views are provided. The anchoring of the director field at the walls is normal for a – d and planar for e – h . Structures correspond to ( a ) and ( e ) w =0.23 and ϕ =1%; ( b ) and ( f ) w =0.23 and ϕ =4%; ( c ) and ( g ) w =2.3 and ϕ =1%; ( d ) and ( h ) w =2.3 and ϕ =4%. As in Fig. 1 , only one quarter of the simulation box is shown for clarity (its horizontal extent being and vertical extent in the narrow direction); the full structures are shown in Supplementary Figs 5 and 6 . Full size image Figure 2e–h shows comparable simulations for planar wall anchoring. Without colloidal particles, planar anchoring results in a regular cholesteric helix, with axis perpendicular to the boundary walls. This twisted texture develops via a set of defect loops, which shrink and disappear to leave a defect-free sample. However, dispersing particles with small w arrests the loop shrinking process, stabilizing twisted rings ( Fig. 2e ) at small ?, and more complicated double-stranded structures at larger ϕ ( Fig. 2f ). For larger w , we observe thick colloidal ‘ropes’ about five particles across ( Fig. 2g,h ). These ropes undulate to follow the chiral structure of the underlying fluid. On increasing the density, they develop branch points and finally again approach a percolating gel morphology. Note that planar wall anchoring is incompatible with the normal anchoring on the colloidal particles (for w >0), which are thus repelled from both walls (see the side views in Fig. 2e–h ). The degree of similarity between the bulk and confined structures is somewhat masked by the local change in particle density in the confined case. If one allows for this, Figs 1 and 2 show that the individual structural motifs are actually rather similar: templated lines for weak anchoring and clusters for strong anchoring. Switching in electric field An interesting question, relevant for applications to devices, is whether these structures can be modified, or switched, with electric fields. 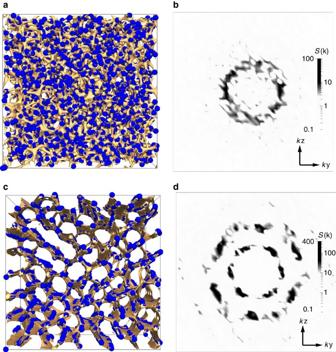Figure 3: Structure in electric field. Steady states obtained when a dispersion of colloids is inserted into a thermodynamically stable bulk BPIII with and without applied external electric field. Panelashows the situation in zero field, and panelcthe situation when the applied field is in thex-direction (perpendicular to the plane of the paper). Panelsbanddshow one plane of the three-dimensional structure factorS(k) computed from the positions of the particles, with wavevectorkx=0, corresponding toaandc, respectively. With field, the disclinations form a honeycomb pattern with hexagonal ordering perpendicular to the field direction; this is reflected in the structure factor. Simulations use weakly anchoring particlesw=0.23 and a volume fraction ofϕ=5% (seeSupplementary Notesfor full list of parameters). The full simulation with a box size ofis shown. Figure 3 addresses this question, starting from amorphous BP III, this time at a higher chirality. Dispersing colloidal particles in this network results in the particle occupying the available nodes, where the order parameter is low ( Fig. 3a ; Supplementary Movie 5 ). Applying a high enough field along the x direction leads to a switching to a new phase, where colloidal arrays fit within a network with distorted hexagonal cells ( Fig. 3b and Supplementary Fig. 7 ; Supplementary Movie 6 ). Remarkably, on field removal this honeycomb structure does not find its way back to the configuration before switching on the field, but gets stuck into a metastable structure ( Supplementary Fig. 7 ), with residual anisotropy along the field switching direction. Cycling the field along the x and y directions leads to distinct metastable structures, which are retained after field removal ( Supplementary Figs 8 and 9 ). We note that for the fluid parameters used here, the field-induced changes are irreversible with the weakly anchoring colloid particles. The mesophase without colloid particles undergoes a reversible ordering transition [10] ; the reversibility is retained in the presence of particles only if their anchoring is very weak. Figure 3: Structure in electric field. Steady states obtained when a dispersion of colloids is inserted into a thermodynamically stable bulk BPIII with and without applied external electric field. Panel a shows the situation in zero field, and panel c the situation when the applied field is in the x -direction (perpendicular to the plane of the paper). Panels b and d show one plane of the three-dimensional structure factor S ( k ) computed from the positions of the particles, with wavevector k x =0, corresponding to a and c , respectively. With field, the disclinations form a honeycomb pattern with hexagonal ordering perpendicular to the field direction; this is reflected in the structure factor. Simulations use weakly anchoring particles w =0.23 and a volume fraction of ϕ =5% (see Supplementary Notes for full list of parameters). The full simulation with a box size of is shown. Full size image The surprising wealth of colloidal-BP composites obtained in Figs 1 , 2 , 3 is the complex consequence of a simple competition between two self-assembly principles. First, BPs provide a three-dimensional template onto which colloidal particles are attracted so as to reduce the elastic stresses arising at the disclination cores [17] . Second, colloidal intrusions in a liquid crystal raise the free energy locally; sharing this cost creates a generic tendency to aggregate into clusters [4] . Which of these factors dominates depends on w , a dimensionless measure of the anchoring strength of the director field at the colloidal surface. For , the templating principle dominates. Colloidal crystals, gels or twisted rings can then arise. For , interparticle attractions defeat the templating tendency, and we predict disconnected aggregates, percolating gels or helical colloidal ropes. In both cases, control is offered by the process route, colloidal concentration and the anchoring conditions at sample walls. We have also shown that electric fields can be used to switch between metastable states, providing a possible route to future multistable device applications. How do these simulations relate to experiment? Several authors have used nanoparticles in the context of stabilizing BPs [32] , [33] . These nanoparticles are typically a few nanometres in size, in which case stabilization is explained by the mechanism of defect removal. Experiments suggest this mechanism is also relevant for larger particles in the range of 40–70 nm (ref. 34 ), which is consistent with the current simulations. However, the mechanism is observed to be less efficient for particles above 100 nm, where particles may start to disrupt longer-range liquid crystal order [34] . While the field of self-assembly with nanoparticles is relatively new [35] , nanoparticles have also been used in both nematic [36] and chiral liquid crystals [37] as host fluid templates. The variation of structure seen in our simulations suggest that some careful characterization of parameters such as surface anchoring of particles (which are often stabilised, or even functionalised with surface ligands), together with those associated with any confining surfaces or interfaces, is required to understand the final structure and to be able to reproduce it with a given experimental protocol. The identification of a model system that could allow unambiguous comparison between experimental systems and simulation would be extremely useful. Such a system might adopt particles of diameter in the range 50 nm or above, which allows a coarse-grained simulation approach of the type used here to be adopted, which can then capture the large-scale structure required to compare with experiment. In the same vein, detailed surface chemistry is difficult to represent in coarse-grained simulations, so heavily functionalized particles might be avoided. We have not explored in this work switchability by flow [38] , but this could again be inherited from the underlying BP dynamics [19] , [28] , in which case the same materials may also be relevant to the emerging technology of optofluidics [39] . Thermodynamics The thermodynamics of the cholesteric liquid crystal can be described by means of a Landau-de Gennes free energy functional , whose density is written as f : This free-energy density f = f ( Q ) may be expanded in powers of the order parameter Q and its gradients; Q is a traceless and symmetric tensor, which is denoted from now on in subscript notation as Q αβ . The largest eigenvalue q and corresponding eigenvector n α of Q αβ describe the local strength and major orientation axis of molecular order. The theory based on the tensor Q αβ , rather than a theory based solely on the director field n α ( r ), allows treatment of disclinations (defect lines) in whose cores n α is undefined. Explicitly, the-free energy density is: Here, repeated indices are summed over, while terms of the form Q αβ 2 should be expanded to read is the permutation tensor. The first three terms are bulk free-energy density whose overall scale is set by A 0 (discussed further below); is a control parameter related to a reduced temperature. Varying the latter in the absence of chiral terms ( q 0 =0) gives an isotropic-nematic transition at with a mean-field spinodal instability at . The remaining two terms of the free-energy density in equation (2) describe distortions of the order parameter field. In theoretical work and when describing a generic rather than a specific system, it is conventional [9] , [40] to assume that splay, bend and twist deformations of the director are equally costly, that is, there is a single elastic constant K . The parameter q 0 is related to the helical pitch length p via q 0 =2 π / p , describing one full turn of the director in the cholesteric phase. There are two dimensionless numbers, which are commonly referred to as κ , the chirality, and τ , the reduced temperature [9] , which can be used to characterize the system. In terms of the parameters in the free-energy density, these are: If the free-energy density (equation (2)) is made dimensionless, τ appears as prefactor of the term quadratic in Q αβ , whereas κ quantifies the ratio between bulk and gradient free-energy terms. The chirality and reduced temperature may be used to characterize an equilibrium phase diagram of the BPs in bulk cholesteric liquid crystals [9] , [21] . The effect of an electric field can be modelled by including the following term in the bulk free-energy density: where E α are the components of the electric field, and (here assumed positive) is the dielectric anisotropy of the liquid crystal. The strength of the electric field is quantified via one further dimensionless number The quantity is known as the reduced field strength. Surface free energy In addition to the fluid free energy density f ( Q αβ ), a surface free energy density is also present to represent the energetic cost of anchoring at a solid surface. In the case of normal anchoring, the surface free-energy density (per unit area) is where is the preferred order parameter tensor at the solid surface, and W is a constant determining the strength of the anchoring. In the case of planar anchoring, a slightly more complicated expression is required to allow for degeneracy (see, for example, ref. 41 ). The determination of for normal and planar anchoring is discussed below. For a colloidal particle of radius R , the strength of the surface anchoring compared with the bulk fluid elastic constant may be quantified by the dimensionless parameter WR / K . For small values of this parameter, the presence of a particle surface should have little impact on the local fluid LC ordering. Dynamics of the order parameter A framework for the dynamics of liquid crystals is provided by the Beris-Edwards model [42] , in which the time evolution of the tensor order parameter obeys In the absence of flow, equation (8) describes a relaxation towards equilibrium on a timescale determined by a collective rotational diffusion constant Γ. This relaxation is driven by the molecular field H αβ , which is the functional derivative of the free energy with respect to the order parameter [42] : The tensor S αβ in equation (8) completes the material derivative for rod-like molecules [42] . It couples the order parameter to the symmetric and antisymmetric parts of the velocity gradient tensor W αβ ≡ ∂ β u α . The symmetric part A αβ and the antisymmetric part Ω αβ are defined as and This full coupling term is then Here, ξ is a material dependent that controls the relative importance of rotational and elongational flow for molecular alignment, and determines in practice how the orientational order responds to a local shear flow. In all cases, the value used here is ξ =0.7, which is within the ‘flow aligning’ regime, where molecules align at a fixed angle (the Leslie angle) to the flow direction in weak simple shear [40] . The value of the collective rotational diffusion used in all simulations is Γ=0.5 in simulation units. Hydrodynamics The momentum evolution obeys a Navier-Stokes equation driven by the divergence of a generalized stress P αβ : The pressure tensor P αβ is, in general, asymmetric and includes both viscous and thermodynamic components: A lattice Boltzmann flow solver is used, where the isotropic pressure p 0 and viscous terms are managed directly by the solver (as in a simple Newtonian fluid, of viscosity η ), whereas the divergence of the remaining terms is treated as a local force density on the fluid. In all simulations reported the mean fluid density ρ =1 and the viscosity η =0.01 (simulations in confined geometry also used enhanced bulk viscosity ζ=10 η to ensure numerical stability). Surface boundary conditions for particles Hydrodynamic boundary conditions for solid objects are handled via the lattice Boltzmann solver. In particular, the standard method of bounce-back on links is used for both particles and confining walls [43] , [44] . Boundary conditions for the order parameter are set out in ref. 45 . In all the simulations reported here the preferred orientation of the director field at the particle surface is normal to the surface. The required nematic director at the particle surface in a given location may then be determined from geometry alone, and a preferred order parameter is computed via The magnitude of surface order q 0 is set by that corresponds to the bulk order in a defect-free nematically ordered sample [46] (this is also very close to the value of the order parameter in a cholesteric or in a BP away from disclinations). In all simulations, the colloidal (hard sphere) radius is R =2.3. To prevent particles overlapping at the hard sphere radius, an additional short range soft potential is included. This takes the form of where h is the surface to surface separation. The parameters are and σ =0.1 in simulation units. Both potential and resulting force are smoothly matched to zero at a cutoff distance of h c =0.25 simulation units. Surface boundary conditions for walls The confining solid walls, which are flat and stationary, have the same normal boundary condition as at the particle surface. In addition, degenerate planar anchoring is applied at the walls, where the preferred nematic director may adopt any orientation parallel to the surface. The preferred direction is determined explicitly by projecting the local fluid order parameter to the plane of the wall [41] . Equation (15) and equation (16) are then used as before. To prevent the particles being forced into the wall, a correction to the lubrication force on the colloidal particle is added for very low particle surface to wall surface separations h <0.5 lattice spacing. The correction is based on the analytic expression for the lubrication between a sphere and a flat surface. How to cite this article: Stratford, K. et al. Self-assembly of colloid-cholesteric composites provides a possible route to switchable optical materials. Nat. Commun. 5:3954 doi: 10.1038/ncomms4954 (2014).